A Polymerase Theta-dependent repair pathway suppresses extensive genomic instability at endogenous G4 DNA sites Genomes contain many sequences that are intrinsically difficult to replicate. Tracts of tandem guanines, for instance, have the potential to adopt stable G-quadruplex structures, which are prone to cause genome alterations. Here we describe G4 DNA-induced mutagenesis in Caenorhabditis elegans and identify a non-canonical DNA break repair mechanism that generates deletions characterized by an extremely narrow size distribution, minimal homology of exactly one nucleotide at the junctions, and by the occasional presence of templated insertions. This typical mutation profile is fully dependent on the A-family polymerase Theta, the absence of which leads to profound loss of sequences surrounding G4 motifs. Theta-mediated end-joining prevails over non-homologous end joining and homologous recombination and prevents genomic havoc at replication fork barriers at the expense of small deletions. G4 DNA-induced deletions also manifest in the genomes of wild isolates of C. elegans , indicating a protective role for this pathway during evolution. To preserve the integrity of genetic information, DNA replication needs to be accurate but also very efficient, as the entire cellular DNA needs to be duplicated before chromosomes can reliably be segregated to the two daughter cells during mitosis. DNA damage, as well as alternative DNA structures that obstruct replication fork progression, thus represents threats to chromosome integrity and to the faithful inheritance of genomes. One non-Watson–Crick DNA structure that is thermodynamically very stable under physiological conditions is a so-called G-quadruplex ( Fig. 1a ). While guanine-rich single-stranded DNA can readily adopt such a structure in vitro , its in vivo formation has remained a subject of debate ever since the structure was first described [1] . Recent years have, however, seen a greatly increased interest in G-quadruplexes due to new insights into their possible roles in various biological processes such as gene expression, epigenetic regulation, telomere maintenance and DNA replication initiation [2] , [3] , [4] , [5] , [6] , [7] , [8] . While genome-wide in silico analyses have identified more than 300,000 G4 motifs (sites with G-quadruplex-forming potential) in the human genome [9] , perhaps the best in vivo evidence thus far for a functional role of G4 DNA comes from the bacterium Neisseria gonorrhoeae . This human pathogen evades its host’s immune system by changing the identity of its surface antigen via a G4 DNA-induced recombination event [10] . Importantly, however, this example also illustrates the recombinogenic and thus potentially pathological nature of this highly thermal stable non-B-DNA structure—a concern further fuelled by the notion of hampered DNA replication near G4 sequences in yeast [11] , [12] , [13] and the observed association of G4 motifs with structural genomic variations in human cancers [14] . 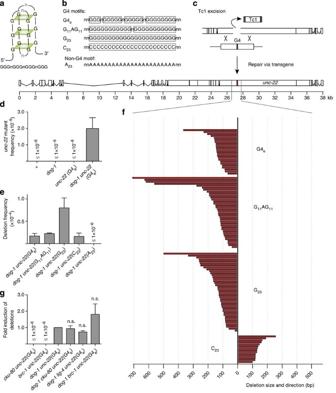Figure 1: A novel genomic selection-based assay to measure G4 DNA instability. (a) Schematic representation of a G-quadruplex structure. (b) DNA sequences that were targeted to the endogenousunc-22locus. The guanines that can participate in the formation of a G-quadruplex structure are boxed. (c) Schematic representation of the targeting strategy in which a Tc1 transposon-induced double-strand break in theunc-22locus is allowed to repair via an extrachromosomal array carrying ~3 kbunc-22sequences interspersed with a G4 motif. The intervening sequence was designed to result in a functionalunc-22ORF upon integration. (d)dog-1- and G4 DNA-dependent mutation induction for the endogenousunc-22. The frequency is based on ±40 independent populations per genotype; the mean of at least two experiments is shown. Error bars indicate s.e.m. (e) Comparison of G4 DNA-induced deletion frequencies at theunc-22locus for different G4 sequence motifs. The frequency is based on ±40 independent populations per genotype; the mean of at least two experiments is shown. Error bars indicate s.e.m. (f) Graphic illustration of the G4 deletion profiles of different G4 motifs; each bar represents one mutant. (g) G4 DNA-induced deletion frequencies for the indicated genetic backgrounds. The fold induction with respect todog-1 unc-22(G4e) is represented, and is based on at least two independent experiments. Error bars indicate s.e.m. No significant (n.s.) difference was found betweendog-1single and double mutants (paired two-tailedt-test). Figure 1: A novel genomic selection-based assay to measure G4 DNA instability. ( a ) Schematic representation of a G-quadruplex structure. ( b ) DNA sequences that were targeted to the endogenous unc-22 locus. The guanines that can participate in the formation of a G-quadruplex structure are boxed. ( c ) Schematic representation of the targeting strategy in which a Tc1 transposon-induced double-strand break in the unc-22 locus is allowed to repair via an extrachromosomal array carrying ~3 kb unc-22 sequences interspersed with a G4 motif. The intervening sequence was designed to result in a functional unc-22 ORF upon integration. ( d ) dog-1 - and G4 DNA-dependent mutation induction for the endogenous unc-22 . The frequency is based on ±40 independent populations per genotype; the mean of at least two experiments is shown. Error bars indicate s.e.m. ( e ) Comparison of G4 DNA-induced deletion frequencies at the unc-22 locus for different G4 sequence motifs. The frequency is based on ±40 independent populations per genotype; the mean of at least two experiments is shown. Error bars indicate s.e.m. ( f ) Graphic illustration of the G4 deletion profiles of different G4 motifs; each bar represents one mutant. ( g ) G4 DNA-induced deletion frequencies for the indicated genetic backgrounds. The fold induction with respect to dog-1 unc-22(G4 e ) is represented, and is based on at least two independent experiments. Error bars indicate s.e.m. No significant (n.s.) difference was found between dog-1 single and double mutants (paired two-tailed t -test). Full size image G4 DNA-induced genomic alterations were first identified in C. elegans , where the DOG-1/FANCJ helicase [15] was shown to suppress deletions initiated at G-rich DNA sequences [16] . Later work demonstrated that only G-rich DNA sequences that match the signature G4 motif G 3–5 N 1–3 G 3–5 N 1–3 G 3–5 N 1–3 G 3–5 define sites of genomic instability [17] ; G-rich DNA unable to adopt a G-quadruplex structure remained perfectly stable in DOG-1-deficient worms. An evolutionary conserved role for DOG-1/FANCJ in preventing G4 DNA-induced genome alteration was suggested by the mapping of large genomic deletions accumulating in a FANCJ-deficient human patient cell line to G4 DNA-containing regions [18] . In line with a proposed role for this helicase in resolving G-quadruplexes in vivo to help the fork replicate the affected strand [16] , the purified human FANCJ protein was shown to behave as a structure-specific DNA helicase that can unwind G4 DNA with 5′ to 3′ polarity [19] . While the molecular nature of genomic alterations in C. elegans demonstrated a strikingly atypical mutation profile [16] , [17] , little is known about the molecular mechanisms that underlie G4 DNA-induced genome rearrangements. Here we identify an alternative DNA double-strand break (DSB) repair pathway, which requires Polymerase Theta (θ), and which is the pathway of choice to cope with these structural replication fork barriers. An endogenous target to monitor G4 DNA instability To investigate the mutagenic mechanism responsible for the generation of deletions at G4 sequences, we first engineered the C. elegans genome to create a selectable system for G4 DNA-induced mutations. Via transposon-mediated insertional mutagenesis [20] , we targeted several distinct G4 motifs to the coding region of the endogenous unc-22 locus, which itself is devoid of G4 motifs. The inserted G4 DNA sequences did not perturb its host reading frame or function ( Fig. 1b,c ). With its 22-kb open reading frame (ORF) and a clearly recognizable mutant phenotype, the unc-22 locus provides an endogenous mutational sink that is largely non-discriminatory to size: all alterations that change the reading frame (whether one bp or tens of kb) will render worms insensitive to the muscle hyper-contracting effect of the cholinergic agonist levamisole [21] . Earlier work revealed that sequences that match the G4 DNA consensus G 3-5 N 1-3 G 3-5 N 1-3 G 3-5 N 1-3 G 3-5 induce deletions in dog-1- deficient animals; equienergetic G-rich DNA sequences that do not match this motif (for example, G3C DNA or CG repeats) are perfectly stable [17] . However, because of the relatively high, size-related, background level of spontaneous mutagenesis in unc-22 (~10 −6 ), we chose to target only those G4 sequences that we previously found to have high mutagenic potential ( Fig. 1b ). Figure 1d demonstrates that a single G4 motif does not profoundly elevate the spontaneous mutation rate in unc-22 in wild-type animals. However, the mutation rate increases ~15–65-fold when introduced into a dog-1 -deficient background, with the fold increase depending on the nature of the G-tract ( Fig. 1d,e ). We found the mutagenicity of the G4 motifs to be dependent on both the G4 sequence and the genomic context: a G 23 monotract was a more potent inducer of deletions than non-monoG G4 sequences, whereas simply changing the polarity of the G 23 tract with respect to the direction of the unc-22 locus dampened its mutagenic potential, indicating that the mutagenic potential is not solely dictated by the nucleotide composition of the G4 motif. Molecular characteristics of G4 DNA-induced genome alterations To determine the features of G4 DNA-induced mutagenesis, we systematically characterized large numbers of mutants ( Figs 1 and 2 , Supplementary Table 1 ). These profiles augment and further refine previously determined deletion characteristics but importantly also lead to novel insight hinting towards an error-prone repair mechanism that generates these deletions. 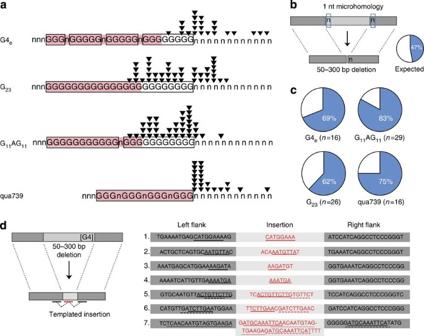Figure 2: Molecular characteristics of G4 DNA-induced deletions. (a) Position of the 3′ junctions with respect to the cognate G4 motif (boxed). Triangles indicate junctions of separately isolated deletion alleles. For each motif, the minimal 5′ sequence that complies to the G4 motif consensus is shown in pink to visually emphasize the notion that almost all junctions (94%) map 3′ of a possible G4 structure. (b) Illustration defining single-nucleotide homology. The chance that the outermost nucleotide on one deletion junction is identical to the first deleted base at the other junctions was calculated as well as empirically determined to be 47% (Supplementary Fig. 1). (c) Pie charts displaying the overrepresentation of single-nucleotide homology for G4 DNA-induced simple deletions (in blue). (d) Templated insertions coinciding with G4 DNA-induced deletion formation. On the left this phenomenon is graphically represented. The right panel displays seven examples. Matching sequences are underlined. Lines 1–4 are simple inserts templated on the 5′ flank. Lines 5 and 6 represent cases where the same flank is used twice as a template. Line 7 represents a case where both the 5′ and 3′ flanks contribute to the insert but also illustrates that the flank 3′ to the G-tract can serve as a template (seeSupplementary Figs 2 and 4for more cases). Figure 2: Molecular characteristics of G4 DNA-induced deletions. ( a ) Position of the 3′ junctions with respect to the cognate G4 motif (boxed). Triangles indicate junctions of separately isolated deletion alleles. For each motif, the minimal 5′ sequence that complies to the G4 motif consensus is shown in pink to visually emphasize the notion that almost all junctions (94%) map 3′ of a possible G4 structure. ( b ) Illustration defining single-nucleotide homology. The chance that the outermost nucleotide on one deletion junction is identical to the first deleted base at the other junctions was calculated as well as empirically determined to be 47% ( Supplementary Fig. 1 ). ( c ) Pie charts displaying the overrepresentation of single-nucleotide homology for G4 DNA-induced simple deletions (in blue). ( d ) Templated insertions coinciding with G4 DNA-induced deletion formation. On the left this phenomenon is graphically represented. The right panel displays seven examples. Matching sequences are underlined. Lines 1–4 are simple inserts templated on the 5′ flank. Lines 5 and 6 represent cases where the same flank is used twice as a template. Line 7 represents a case where both the 5′ and 3′ flanks contribute to the insert but also illustrates that the flank 3′ to the G-tract can serve as a template (see Supplementary Figs 2 and 4 for more cases). Full size image First, we establish that the previously observed atypical and strikingly narrow deletion size distribution is intrinsic to G4 DNA instability; while the G4 motifs are located in a largely size non-discriminatory locus, 92% of deletions (104 out of 113) are between 50 and 300 bp, with only nine cases being shorter or longer—the shortest being 14 bp and the longest being 704 bp ( Fig. 1f ). The nucleotide composition of the G4 motif does not significantly affect deletion size: median sizes being 137 bp, 128 bp, 123 bp and 128 bp for G4 e , G 11 AG 11 , G 23 and C 23 , respectively. Second, we strengthen the suggestion that the premutagenic lesion is in fact a quadruplex fold. While all deletions have their 3′ junction close to the start of the G4 motif, the exact position is greatly influenced by the exact sequence of the motif; whereas the 3′ junctions of deletions induced by the sequence G4 e centres around the outermost G of the G4 motif, the 3′ junctions at G 23 and G 11 AG 11 are located more internally ( Fig. 2a ). This increased spread is in line with the notion that the latter motifs are able to adopt many different quadruplex conformations that satisfy the G-quadruplex consensus G 3–5 N 1–3 G 3–5 N 1–3 G 3–5 N 1–3 G 3–5 . A quadruplex fold comprising only the 15 5′ guanines of a G 23 monotract would allow replication to progress through eight 3′ guanines before being blocked, ultimately resulting in a junction positioned within the tract. We further tested whether the first blocking guanine of a quadruplex fold determines the position of the 3′ deletion junction by establishing via polymerase chain reaction (PCR) a 3′ junction profile for a minimal G4 tract, qua739: GGGtGGGaGGGtGGG, which can adopt only one possible three-stacked quadruplex configuration (see Fig. 1a ). As of the low mutagenic capacity of minimal G4 motifs [17] , we obtained qua739 deletions at its original genomic location using a PCR-based approach (see Methods section). Indeed, deletions triggered by this motif have a very sharply positioned 3′ junction, with none mapping within the motif ( Fig. 2a ). We then unexpectedly found that also the position of the 5′ junction is not random, and in fact is linked to the nucleotide composition of the 3′ junction. At first glance, the 5′ junctions appeared evenly distributed over a 50- to 300-bp region upstream of the G4 motif, without any preferential site or sequence ( Fig. 1f ). However, upon close examination, we observed what could be termed as single-nucleotide homology: ~60–80% of the 81 simple deletions (without inserts) had at least one nucleotide that could be mapped to either junction ( Fig. 2b,c ), which is profoundly more than the 47% chance if the deletions would be randomly distributed or when compared with a randomly generated set of ~18,000 deletions ( P <0.0001, χ 2 test; see Supplementary Fig. 1 for details). This overrepresentation is not restricted to deletions induced by G4 motifs at the unc-22 locus; by whole-genome sequencing of three dog-1 strains that have been clonally grown for 50 generations, we found 59 unique simple deletions mapping to different genomic G4 motifs, 73% of which have homology at their most terminal nucleotide ( P <0.0001, χ 2 test, Supplementary Fig. 2 , Supplementary Table 2 ). This phenomenon that may suggest the use of microhomology can, however, be completely attributed to the first nucleotide; while the greatly increased level of homology at the terminal position is highly significant, this is not the case for the neighbouring bases. In fact, in more than 40% of the simple deletions, the homology is restricted to a single nucleotide; the number of observed cases having two bases of microhomology is statistically not different from a random distribution ( P =0.3, χ 2 test), taken into account the increased incidence of one nucleotide homology. This fact, together with the notion that more prominent sequence homology can frequently be found in the immediate vicinity of the 5′ junctions, argues that homology itself is not a driving force in the molecular events leading to deletion formation. Instead, we envisage this single-nucleotide homology to reflect the action of a DNA polymerase acting on and extending a one-base-pair intermediate in an alternative end-joining repair mechanism. The observation that genetically inactivating non-homologous end joining or HR affected neither G4 DNA-induced mutation rate nor spectra ( Fig. 1g , Supplementary Fig. 3 and the study by Kruisselbrink et al . [17] ) supports this hypothesis. Another novel characteristic that points towards the involvement of a DNA polymerase is the presence of insertions accompanying 28% of all unc-22 deletions (32/113). For cases where insertions are larger than four nucleotides, their origin can be traced back to the sequence immediately flanking the junction ( Fig. 2d , Supplementary Figs 2 and 4 , Supplementary Tables 1 and 2 ). While many inserts map 5′ to the G-tract, we also found cases where newly inserted DNA matched the 3′ flank ( Fig. 2d , line 7; Supplementary Figs 2 and 4 , Supplementary Tables 1 and 2 ), suggesting that a free 3′ extendable end is available at either side of the G-tract. The latter observation is important because it argues for the existence of a DNA DSB as an intermediate in the generation of deletions at G4 DNA sites, a conclusion that is strengthened by an increased number of foci of the DSB marker RAD-51 observed in both germ and somatic cells in dog-1 animals, as compared with wild-type animals ( Supplementary Fig. 5 ). Two observations suggest that the 3′ ends of these breaks are fairly stable and refractory to trimming; first, templated inserts were typically found very close to their cognate template, suggesting that newly made DNA was joined to the DNA that served as its template, and second, we found cases in which the same flanking sequence was used as a template twice consecutively ( Fig. 2d , lines 5–7; Supplementary Fig. 2 ), indicative of iterative cycles of extension and repriming. The typical G4 DNA-induced deletions require polymerase θ After having established the signature of polymerase activity in G4 DNA-induced deletions, we set out to identify the responsible DNA polymerase via a candidate approach. We assayed mutants of the translesion synthesis polymerases η and κ, as these Y-family polymerases have the ability to replicate through damaged DNA and have previously been suggested to play a role in G4 DNA-mediated deletion induction [22] . We found, however, no evidence for their involvement using multiple approaches and combinations of alleles ( Table 1 , Supplementary Fig. 6a,b ). Table 1 Quantification G4 DNA-induced deletions using PCR assays. Full size table Another candidate is polymerase θ, an A-family DNA polymerase implicated in the repair of interstrand crosslinks [23] , [24] , [25] . Mammalian Pol θ has the ability to bypass DNA lesions and to extend matched as well as mismatched primer termini [26] , [27] . In addition, Drosophila Pol θ was recently implicated in the repair of DNA DSBs induced by DNA transposition [28] . To test a possible involvement of the C. elegans homologue of Pol θ, POLQ-1, we first used a PCR-based assay that detects G4 DNA-induced deletions in isolated DNA by preferential amplification of smaller than wild-type bands of sequences containing G4 motifs [17] . We found that, while 14% of dog-1 animals sustained at least one small-sized deletion at the G4 motif qua830, none were detected in animals that in addition were also deficient for polq-1 ( Fig. 3a ). The same outcome was found for different G4 DNA-containing loci, and when different alleles of dog-1 and polq-1 were tested ( Table 1 , Supplementary Fig. 6c ), together indicating that deletion induction at endogenous G4 motifs is completely dependent on functional POL θ. 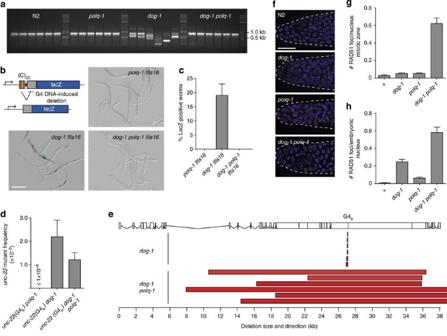Figure 3: Polymerase Theta-mediated end-joining G4 DNA-induced DNA breaks. (a) PCR-based assay to measure G4 DNA-induced deletion formation. Animals of the indicated genotype (five per lane) are lysed and PCR-amplified with primers flanking the endogenous G4 motif, qua830. Somatic deletions will manifest as shorter than wild-type product (which is present in great excess). (b) Reporter-based assay to measure G4 DNA-induced deletion formation using LacZ expression as read out. The panels display 5–10 animals stained for LacZ and their indicated genotypes. SeeMethodssection for detailed description of reporter and assay. Scale bar indicates 0.25 mm. (c) Quantification of reporter LacZ expression by scoring animals (n>200 per experiment) of the indicated genotype for the presence of1 blue cell. The average percentage of at least four independent experiments is shown. Error bars indicate s.e.m. (d) Mutation frequency at the genomicunc-22(G4e) allele for the indicated genotypes. The frequency is based on ±50 independent populations per genotype; the mean of at least two experiments is shown. Error bars indicate s.e.m. (e) Graphical representation of theunc-22mutations isolated from the indicated genotype. Bars represent the size and location of independently derivedunc-22deletions. (f) Immunohistochemical analysis of proliferative germ cells in the mitotic zone of theC. elegansgonad. RAD-51 foci in red; 4',6-diamidino-2-phenylindole in blue. Scale bar indicates 15 μm. (g,h) Quantification of RAD-51 foci in the proliferative pre-meiotic germline,n14 germlines per genotype (g) and in developing embryos,n18 embryos per genotype (h). (a–h) N2,dog-1(gk10)andpolq-1(tm2026)alleles were used; error bars indicate s.e.m. Figure 3: Polymerase Theta-mediated end-joining G4 DNA-induced DNA breaks. ( a ) PCR-based assay to measure G4 DNA-induced deletion formation. Animals of the indicated genotype (five per lane) are lysed and PCR-amplified with primers flanking the endogenous G4 motif, qua830. Somatic deletions will manifest as shorter than wild-type product (which is present in great excess). ( b ) Reporter-based assay to measure G4 DNA-induced deletion formation using LacZ expression as read out. The panels display 5–10 animals stained for LacZ and their indicated genotypes. See Methods section for detailed description of reporter and assay. Scale bar indicates 0.25 mm. ( c ) Quantification of reporter LacZ expression by scoring animals ( n >200 per experiment) of the indicated genotype for the presence of 1 blue cell. The average percentage of at least four independent experiments is shown. Error bars indicate s.e.m. ( d ) Mutation frequency at the genomic unc-22 (G4 e ) allele for the indicated genotypes. The frequency is based on ±50 independent populations per genotype; the mean of at least two experiments is shown. Error bars indicate s.e.m. ( e ) Graphical representation of the unc-22 mutations isolated from the indicated genotype. Bars represent the size and location of independently derived unc-22 deletions. ( f ) Immunohistochemical analysis of proliferative germ cells in the mitotic zone of the C. elegans gonad. RAD-51 foci in red; 4',6-diamidino-2-phenylindole in blue. Scale bar indicates 15 μm. ( g , h ) Quantification of RAD-51 foci in the proliferative pre-meiotic germline, n 14 germlines per genotype ( g ) and in developing embryos, n 18 embryos per genotype ( h ). ( a – h ) N2, dog-1(gk10) and polq-1(tm2026) alleles were used; error bars indicate s.e.m. Full size image We next visualized G4 DNA instability directly in animals using transgenes that express LacZ when a G4 DNA-induced deletion brings the reporter ORF in frame with the upstream ATG start codon ( Fig. 3b ). Twenty percent of dog-1 -deficient animals stochastically express LacZ in various cell types with patterns indicative of G4 DNA-induced deletion events occurring at different stages of embryonic development ( Fig. 3b ). In contrast, no LacZ-expressing cells were observed in dog-1 polq-1 -mutant animals, again indicating that the generation of the characteristic asymmetrical 50- to 300-bp deletions at G4 motifs is completely dependent on POL θ functionality ( Fig. 3b,c ). Apart from null alleles of polq-1 , we also tested an allele (generated via random mutagenesis in the C. elegans million mutation project [29] ) that has a mutation in its polymerase domain. A change of an evolutionarily highly conserved proline residue at position 1417 into a serine (P1417S) led to a 50% reduction in the number of deletions at endogenous and transgenic G4 sites, which supports a direct role for the polymerase function of POLQ-1 in the generation of G4 DNA-induced deletions ( Supplementary Fig. 7 ). To address the fate of G4 DNA-induced breaks in the absence of functional POL θ, we assayed mutation induction at G4 e within the unc-22 locus. Remarkably, the G4 e -related mutation frequency was only slightly reduced in dog-1 polq-1 animals as compared to dog-1 animals ( Fig. 3d ) indicating that POLQ-1 loss does not affect the mutagenicity of G4 sequences per se . The unc-22 mutants isolated in this genetic background are, however, of a completely different nature; deletions were still observed but were all >10 kb and bidirectional with respect to the G4 motif ( Fig. 3e ). This outcome likely goes together with substantial DNA end resection, as we also observed a profound increase of RAD-51 foci in dog-1 polq-1 double-mutant animals as compared with either single mutant ( Fig. 3f–h , Supplementary Fig. 8 ). G4 DNA instability in natural isolates Thus far, G-quadruplex-induced DNA rearrangements have been observed only in dog-1 -deficient backgrounds; we have not identified events in wild-type animals using five different assays (that is, aCGH, whole genome sequencing, PCR on endogenous loci, unc-22::G4 mutation induction and G4 DNA-reporter transgenes). Given the threshold levels of detection for these assays, we estimated that G4 sequences are at least 1,000-fold more stable in wild type than in dog-1 -deficient animals. We hypothesized that G4 DNA instability may be apparent when analysed on an evolutionary scale and indeed found, by comparative genome analysis of natural isolates of C. elegans ( Fig. 4a ), that G4 DNA-induced deletions occur also during normal growth in genetically non-compromised animals. The Hawaiian strain CB4856 suffered 14 deletions that contained one of the ~1,700 G4 motifs present in the genome of the Bristol N2 strain, from which it is estimated to be ~600,000 generations separated ( Supplementary Table 3 and Methods). In the majority of these cases, the G4 motif is located within few bases of the deletion’s 3′ junction ( Supplementary Table 3 ), a distribution that is highly non-random ( Fig. 4b ). We found another 12 such cases in the genomes of three other natural isolates (CB4857, RC301 and AB2) that are less diverged from Bristol N2 and that live in similar habitats ( Supplementary Table 3 ). Also here, the non-symmetrical deletion fingerprint previously established for dog-1 -deficient animals is apparent ( Fig. 4c ), arguing that G4 DNA-induced deletions in dog-1 and wild-type animals are generated via the same error-prone mechanism. Moreover, these deletions are characterized by single nucleotide homology (69%) and templated insertions (2 out of 17, Fig. 4d ), strongly suggesting that they have been generated via polymerase θ-mediated end joining. 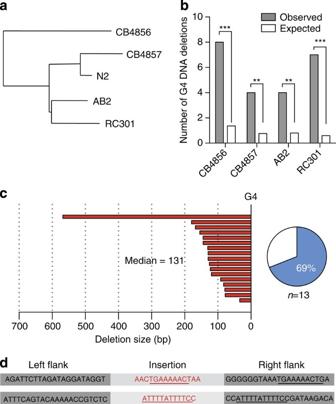Figure 4: G4 DNA instability duringC. elegansevolution. (a) A phylogenetic tree of theC. elegansnatural isolates used in this study, with (b) the observed versus expected number of G4 DNA-induced deletions in their genomes. Bristol N2 was used as a reference genome (seeMethodsfor further details) ***P<1 × 10−5, **P<1 × 10−2, binomial test. (c) Graphic representation (analogous toFig. 1f) of the sizes of the G4 deletions found inC. elegansnatural isolates, the G4 motif is set at 0 (bp). The pie chart displays the overrepresentation of single-nucleotide homology for G4 DNA-induced simple deletions (in blue). (d) Templated insertions coinciding with G4 DNA-induced deletion formation found inC. elegansnatural isolates. Matching sequences are underlined. In both cases the G4 motif was located near the right junction, further strengthening the notion that also the flank 3′ to the G-tract can serve as a template. Figure 4: G4 DNA instability during C. elegans evolution. ( a ) A phylogenetic tree of the C. elegans natural isolates used in this study, with ( b ) the observed versus expected number of G4 DNA-induced deletions in their genomes. Bristol N2 was used as a reference genome (see Methods for further details) *** P <1 × 10 −5 , ** P <1 × 10 −2 , binomial test. ( c ) Graphic representation (analogous to Fig. 1f ) of the sizes of the G4 deletions found in C. elegans natural isolates, the G4 motif is set at 0 (bp). The pie chart displays the overrepresentation of single-nucleotide homology for G4 DNA-induced simple deletions (in blue). ( d ) Templated insertions coinciding with G4 DNA-induced deletion formation found in C. elegans natural isolates. Matching sequences are underlined. In both cases the G4 motif was located near the right junction, further strengthening the notion that also the flank 3′ to the G-tract can serve as a template. Full size image Owing to their ability to obstruct replication fork movement, G-quadruplex structures have recently emerged as DNA sequences at risk for replication fork arrest [12] , [13] and spontaneous chromosomal rearrangements [14] . Whether these structures pose a block to lagging strand synthesis [16] or leading strand synthesis, as was suggested by data derived in yeast [13] , is unknown, and there are no indications in our experiments hinting towards one or the other. We can nevertheless rule out a requirement for ongoing transcription across a G4 locus for it to become mutagenic, as was recently shown to be the case for G4-induced antigenic variation in N. gonorrhoeae [30] : some of the G4-containing loci we studied, including the one in unc-22 , are not transcribed in germ cells [31] ; still they give rise to inheritable genome alterations. Of interest, the inclusion of highly mutagenic G4 sequences, in either orientation, into the coding strand of unc-22 did not affect its expression, which argues that single G4 motifs are not strong modifiers of transcription or translation. Here we show that in C. elegans , a POL θ-dependent pathway acts to prevent extensive loss of sequences near G4 DNA sites but at the expense of generating small deletions. These deletions are typified by a limited size distribution, single-nucleotide homology and the occasional inclusion of templated insertions, and can be recognized in genetic backgrounds that are compromised for their ability to resolve G-quadruplexes through dedicated helicase actions (that is, dog-1 ), as well as in wild-type strains isolated from geographically different regions of the globe. The deletion spectra provide hints as to how POL θ acts to generate deletions of 50–300 bp. The notion of single-nucleotide homology may reflect an extension reaction primed on a one-base-pair intermediate. To us, this interpretation is more plausible than to assume that annealing of a single base provides sufficient stability to seal the breaks by other means. Instead, we propose that POL θ extends this single base pair intermediate, and as such is the creator of extended homology, that is subsequently sufficient to guide break repair. The occasional presence of templated insertions associated with deletion formation may testify to this scenario by reflecting repair false starts, in which an initial primed extension reaction (leading to the incorporation of a number of templated nucleotides) is abrogated, and subsequently restarted by re-annealing and extension, but now at a new position that is defined by the 3′ end of the templated insert ( Fig. 5 ). 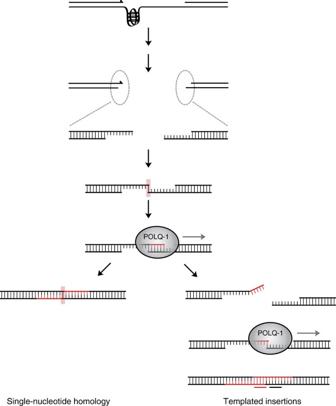Figure 5: Tentative model for polymerase Theta-mediated end joining. A replication fork block at a G4 structure results in a DSB (see alsoSupplementary Fig. 9). The broken ends are joined by polymerase Theta-mediated end joining (TMEJ) resulting in two types of deletions: first, simple ones characterized by single-nucleotide homology, and secondly, deletions with associated templated insertions. The generation of the latter class is simply an iteration of the steps leading to the simple deletions, with one exception being the dissociation of both ends after initial Pol Theta-mediated templated DNA synthesis. Figure 5: Tentative model for polymerase Theta-mediated end joining. A replication fork block at a G4 structure results in a DSB (see also Supplementary Fig. 9 ). The broken ends are joined by polymerase Theta-mediated end joining (TMEJ) resulting in two types of deletions: first, simple ones characterized by single-nucleotide homology, and secondly, deletions with associated templated insertions. The generation of the latter class is simply an iteration of the steps leading to the simple deletions, with one exception being the dissociation of both ends after initial Pol Theta-mediated templated DNA synthesis. Full size image From the nature of the deletion junctions, as well as from the analysis of RAD-51 foci, we infer that POL θ acts to connect DNA ends of DSBs that arise at replication fork barriers. Direct demonstration of these DSBs via molecular means has thus far been unsuccessful, probably because of the very low rates of deletion formation (10 −5 per animal generation). The notion that templated inserts are derived from sequences located both upstream as well as downstream of the G4 argues that extendable 3′ hydroxyl ends are available on either side of the G4, hence a DSB. This notion also disfavours a model in which POL θ would act as a G4 translesion synthesis polymerase by facilitating the nascent G4-blocked strand to jump ahead 50–300 nucleotides, as this would predict that only the sequence ahead of the G4 can act as a template. While current and previous work showed that G4 DNA-induced deletion formation in C. elegans is independent of canonical non-homologous end joining ( Fig. 1g , Supplementary Fig. 3 and studies by Kruisselbrink et al . [17] and Youds et al . [22] ), the outcome is similar: it safeguards genetic integrity by minimizing the loss of genetic information at break sites, via joining the ends. We thus propose to term this alternative end-joining pathway, TMEJ, for polymerase Theta-mediated end joining. Why TMEJ generates deletions specifically in the range 50–300 bp is not known, but may reflect the asymmetric generation of stable free 3′ hydroxyl ends around G-quadruplexes that subsequently serve as substrates for POL θ activity. The nascent strand blocked at the G4 structure provides one obvious point of entry; however, the origin of the more distal end is less clear. Notably, the size distribution of G4 DNA-induced deletions correlates to predicted distances between replication blocks and upstream Okazaki fragments [32] , thus to ssDNA gaps containing a replication fork barrier. Next-round replication of such gaps in rapidly dividing tissues would predict the formation of a DSB with 3′ hydoxyl ends 50–300 bp apart, across from a sister chromatid that still contains the obstructing lesion ( Supplementary Fig. 9 ). Evoking such a scenario for DSB formation may also explain why we thus far failed to find any (structure-specific) nuclease to be required for G4 DNA-induced deletion formation (studies by Kruisselbrink et al . [17] and Youds et al . [22] ; data not shown). The unavailability of the sister chromatid as the preferred repair donor could explain why homologous recombination cannot operate to repair these replication-associated DNA breaks, by that very fact providing the biological raison d’être of TMEJ. Whether TMEJ acts to prevent genomic catastrophe at replication-blocking structures (or lesions) in mammalian systems is an outstanding question that future work needs to address. The outcome of the dynamic interplay between available repair systems can be context- and species-specific, and the notion that expression of mammalian POLQ appears to be highest in testis and human placental tissue [33] may suggest cell lineage-specific use of a POLQ pathway, perhaps favouring error-prone repair over cell death or arrest in situations where rapid cycles of proliferation is critical, as in the C. elegans embryo [34] . We anticipate that ectopic activation of TMEJ may be of high clinical significance, also considering the recent finding that Polymerase Theta upregulation is associated with poor survival in cancer [35] , [36] ; if not properly controlled, POL θ’s ability to tie DNA ends together can have very undesirable effects, as it provides cells with the means to proliferate in the presence of increased replication stress [37] . Blocking this activity may thus constitute a potent strategy towards preventing cancerous growth. Strains and culturing Nematodes were cultured according to standard protocols [21] . The following alleles were used in this study: unc-22(lf39) [G 23 ], unc-22(lf72) [G4 e ], unc-22(lf73) [G 11 AG 11 ], unc-22(lf95) [A 23 ], unc-22(lf96) [C 23 ], dog-1(pk2247) , dog-1(gk10) , rde-2(pk1657) , polk-1(lf29) , polh-1(lf31) , polh-1(ok3317) , cku-80(ok861) , lig-4(ok716), brc-1(tm1145), polq-1(tm2026) , polq-1(tm2572) , polq-1(gk765752), lfIs16[hsp::ATG-C 23 -stops-GFP-LacZ(prp3019);rol-6 D (su1006)], lfIs055 [myo-2::C 23 -stops-GFP-LacZ(pLM20); rol-6 D (su1006)], lfIs177[myo-2::ATG-C 23 -stops-NLS-GFP-LacZ(pLM88); pGH8;pCFJ104;rol-6 D (su1006)] . Alleles were generated in our laboratory or kindly provided by the C. elegans Genetics Center and the laboratory of Dr. Shohei Mitani. Transposon-mediated insertional mutagenesis Cloning details and plasmid sequences are available upon request. In brief, targeting vectors contained G4 sequences flanked by ~1–2 kb of sequence identical to the unc-22 genomic sequence flanking unc-22(st136::Tc1) . Plasmids were co-injected with marker plasmid pRF4 into N2 according to standard protocols. Extrachromosomal arrays were crossed into a mutator background ( rde-2 ) also carrying unc-22(st0136::Tc1) . Populations were screened for unc-22 revertants that were subsequently molecularly analysed. Animals that had reverted because of successful targeting of the G4 sequence to the endogenous unc-22 gene were out-crossed to N2. Unc-22 forward mutation frequency assay The unc-22 forward mutation frequency was determined [38] . In brief, for each data point, 20–100 L4-stage worms were singled on 9-cm plates and grown until the F2–F3 generation. A subfraction of each population was inspected for unc-22 mutants that are resistant to the paralysing effect of (2 mM) levamisole. Independently derived mutants were molecularly analysed using PCR and sequencing. Deletions at endogenous G4 DNA loci Endogenous G4 DNA loci were assayed using a PCR-based approach [39] , [40] . Genomic DNA was isolated either from single worms or pools of worms and subjected to nested rounds of PCRs with primers that flank a G4 motif; amplicons are typically 1 kb in size. Smaller than wild-type bands (deletions) are preferentially amplified (a) because they have the intrinsic bias to amplify small over large DNA segments and (b) because the G4 motif in non-deletion carrying fragments also hamper DNA replication in vitro [39] . To determine the frequency of deletions, L4 stage worms were used (one animal in a 15 μl lysis reaction of which 1 μl was used in a PCR). The following primers were used: qua830 5′-CTAGTTCAGGGTATCTGGAC-3′; 5′-GATTGCGGGCACTTTACCTCG-3′; 5′-CCTTCTCTCGAAGCGCGACC-3′; 5′-GATTTTATTGACTCTCCGTCCG-3′. qua1894 5′-ATTGTGGGAAAAATCCGACG-3′; 5′-TTTGCCATCAAGGTTCCAGAC-3′; 5′-GTATAAGAGTTCCTGGTCGGC-3′; 5′-GGATTTCACAGCGTCAAGAG-3′; qua739 5′-AACGGACAATTATGAGCTACGC-3′; 5′-GATAAGAGAAACGCAAATTACGG-3′; 5′-CCTTGGCTTGGATTTCTTCG-3′; 5′-AAGGCGCACAGATTTTAAGC-3′. LacZ-based transgenic reporter assay Transgenic animals were generated that carry a multicopy array of the reporter construct pRP3019 ( lfIs16 ). pRP3019 was constructed using the backbone of pRP1821 (ref. 41 ). As illustrated in Fig. 3b , a G4 motif (yellow) was placed, in reversed orientation, downstream of the start codon of a heatshock-driven LacZ reporter. Immediately downstream of the tract, stop codons (red) were introduced followed by a non-selective ORF (grey) that is in frame with the LacZ ORF (blue) and functions as a deletion buffer. This reporter will only express LacZ when the stop codons are deleted in vivo —for example, via a typical G4 DNA-induced deletion—and the downstream ORF is brought into frame with the upstream ATG. To read-out G4 DNA instability, lfIs16 animals were synchronized by bleaching and overnight hatching and then transferred to new plates and heat-shocked (34 °C for two times 2 h with 30-min recovering time in between) when animals reached the L3–L4 stage. LacZ expression was visualized with X-gal staining protocol [41] . Experiments were performed at least in triplo for each genotype, each experiment consisting of 4 independent populations having more than 100 worms. G4 DNA reporters pLM20 and pLM88, used to generate alleles lfIs055 and lfIs177 , respectively, deviate slightly from pRP3019 but have the same principle and outcomes. Maps for these reporters are available upon request. Injection marker plasmids pGH8 and pCFJ104 (used for lfIs177 ) are described in the study by Frøkjær-Jensen et al . [42] Immunostainings and RAD-51 foci quantification Germlines were dissected from young adults (1 day post-L4 stage) and processed for immunostaining [43] . Samples were incubated overnight at room temperature with primary anti-RAD-51 antibodies (Novus Biologicals no. 29480002) diluted 1:200 in PBSTB (phosphate-buffered saline with 0.1% Tween 20 and 1% bovine serum albumin), followed by antibody AlexaFluor 488 (Invitrogen no. A11008, diluted 1:1,000 in PBSTB). DNA was stained with 0.5 μg ml −1 4',6-diamidino-2-phenylindole. Samples were mounted with Vectashield. Microscopy was performed with a Leica DM6000 microscope. Whole-genome sequencing of dog-1 mutation accumulation lines dog-1(pk2247) animals were substantially out-crossed to wild-type N2 (Bristol), and mutation accumulation (MA) lines were generated by cloning out F1 animals from one hermaphrodite. Each generation, three worms were transferred to new plates and MA lines were maintained for 50 generations. A single animal was then cloned out and propagated to obtain a full plate for DNA isolation. Worms were rinsed off with M9 and incubated for 1 h at room temperature while shaking. After two washes, worm pellets were lysed for 2 h at 65 °C with SDS containing lysis buffer. Genomic DNA was purified by using a DNeasy kit (Qiagen). Paired-end libraries for whole-genome sequencing (HiSeq2000 Illumina) were constructed from genomic DNA according to the manufacturers’ protocols. The genomes of three independently grown dog-1(pk2247) MA strains were sequenced. Bioinformatic analysis was performed as follows: paired-end whole-genome sequence data of dog-1(pk2247) MA lines were mapped to the reference genome (Wormbase release 225) using bwa with normal settings. Sorted BAM files were created by Samtools and subsequently analysed using Pindel [44] . A deletion was considered only if it was uniquely seen in one of the three sequenced strains and covered at least five times, thereby excluding events that were already present in the starting strain. Raw sequences have been made publicly available at NCBI SRA (Accession code SRP032440). G4 DNA deletions in natural isolates Paired-end whole-genome sequence data were downloaded from the NCBI Short Read Archive (SRP011413), and sequence reads were mapped to the C. elegans reference genome (Wormbase release 225). The average base coverage was 176 × , 164 × , 166 × and 75 × for AB2, CB4857, RC301 and CB4856, respectively. Pindel [44] was used to detect structural variations (SVs) in the natural isolates as compared with the N2 reference genome. We included only SVs that had at least 10 reads supporting the SV and no reads supporting the reference genome. We used the samtools mpileup command to include only those events that showed a coverage drop for the sequence within the SV (average deletion coverage <5x and surrounding flanks (100 bp) coverage >10x). As a third criterion, we collected only those SVs that were N2-like in one of the other three natural isolates. We found 1626, 913, 962 and 714 deletions of at least 10 bp for CB4856, CB4857, AB2 and RC301, respectively. In this collection of SVs, we searched for deletions that contained a G4 motif. We tested seven cases with Sanger sequencing; all of these confirmed the Pindel junction prediction. Statistical analysis We determined the statistical significance of elevated G4 DNA deletion induction in the natural isolates as follows: we first determined the probability of a deletion junction to be within 50 nucleotides of a G4 motif, as 100% of G4 DNA-induced deletions in dog-1 comply to this definition. This probability is 8.4 × 10 −4 : 50 × 1,680 (the number of G4 motifs in the genome)/1 × 10 8 (the size of the genome). The expected number of G4 DNA-induced deletions, as displayed in Fig. 4 , is then set to n × 8.4 × 10 −4 , where n is the total number of deletions found in a strain. We then used binomial distributions to calculate the P- values for the observed number of G4 DNA-induced deletions, given the probability of 8.4 × 10 −4 and the total number of deletions per strain are 1626, 913, 962 and 714 deletions in CB4856, CB4857, AB2 and RC301, respectively. For other experiments, statistical significance was determined with a two-tailed unpaired Student’s t -test, unless otherwise stated. Accession codes: Raw sequences have been made publicly available at NCBI SRA (Accession code SRP032440 ). How to cite this article: Koole, W. et al . A Polymerase Theta-dependent repair pathway suppresses extensive genomic instability at endogenous G4 DNA sites. Nat. Commun. 5:3216 doi: 10.1038/ncomms4216 (2014).